Metabolism of multiple glycosaminoglycans byBacteroides thetaiotaomicronis orchestrated by a versatile core genetic locus The human gut microbiota (HGM), which is critical to human health, utilises complex glycans as its major carbon source. Glycosaminoglycans represent an important, high priority, nutrient source for the HGM. Pathways for the metabolism of various glycosaminoglycan substrates remain ill-defined. Here we perform a biochemical, genetic and structural dissection of the genetic loci that orchestrates glycosaminoglycan metabolism in the organism Bacteroides thetaiotaomicron . Here, we report: the discovery of two previously unknown surface glycan binding proteins which facilitate glycosaminoglycan import into the periplasm; distinct kinetic and genetic specificities of various periplasmic lyases which dictate glycosaminoglycan metabolic pathways; understanding of endo sulfatase activity questioning the paradigm of how the ‘sulfation problem’ is handled by the HGM; and 3D crystal structures of the polysaccharide utilisation loci encoded sulfatases. Together with comparative genomic studies, our study fills major gaps in our knowledge of glycosaminoglycan metabolism by the HGM. The human gut microbiota (HGM) is a vast microbial community that is crucial to human health [1] . The maintenance of the HGM is dependent on its ability to utilise complex glycans as a nutrient source, in the form of dietary and host glycans [2] . The mechanisms by which this community metabolises these glycans is therefore critical to understanding the ecology of the system and how it could be manipulated to benefit human health. Bacteroidetes is one of the two major phyla that dominate the HGM [3] . These organisms dedicate up to 20% of their genome to complex glycan metabolism in the form of genes primarily encoding carbohydrate active enzymes such as, polysaccharide lyases (PLs), glycoside hydrolases, glycan transport and binding proteins, and carbohydrate sulfatases. Bacteroides arrange these genes into polysaccharide utilisation loci (PUL) which are co-localised, co-regulated genes, in response to a specific glycan [4] , [5] . The vast majority of our understanding of how Bacteroidetes metabolise complex glycans is based on dietary plant glycans [6] , [7] , [8] , [9] yet host glycans represent a substantial carbon reservoir, which is also accessed by the HGM [10] , [11] . Glycosaminoglycans (GAGs) have been demonstrated to be a high-priority carbon source for the HGM organism Bacteroides thetaiotaomicron (B. theta) [11] , [12] , and although a pathway for Heparin/Heparan sulfate [13] (H/HS) has been described, the metabolism of the complex, and distinct, GAGs chondroitin sulfate (CS-A and CS-C), dermatan sulfate (DS) and hyaluronic acid (HA) is poorly described. Enzymes of the HGM that metabolise CS have been described [13] , [14] , [15] , yet how they co-ordinate together, their mechanistic details, mode of action and sulfation tolerances remain largely opaque. In addition, the role and mechanism of action of the surface glycan binding proteins (SGBPs) in the degradation of CS, DS and HA is unknown. Here we report how a core PUL has evolved to metabolise the complexity and heterogeneity of CS-A, CS-C, DS and HA. The PUL CS/DS/HA is co-regulated with distant genes, including a hyaluronidase belonging to the recently classified PL33 [16] , to complement its core activities and thus fully enabling multiple GAG breakdown. Crystal structures of the two PUL-encoded carbohydrate sulfatases provide key insights into substrate recognition by these critical, and therapeutically relevant [17] , enzymes. The data enable a general model to be proposed for the metabolism of CS, DS and HA by the HGM and the Bacteroidetes phylum in a wider context. Structure of CS-A, CS-C, DS and HA CS-A and CS-C are both composed of repeating disaccharide units composed of d -glucuronic acid (GlcA) and N-acetyl-D-galactosamine (GalNAc). GlcA is linked β(1,3) to GalNAc which is then linked β(1,4) to the next GlcA. CS-A and CS-C differ only in sulfation with CS-A highly enriched in O4 sulfation on GalNAc whilst CS-C is enriched in O6 sulfation on GalNAc. DS is related to CS-A except GlcA is predominantly replaced with l -iduronic acid which is connected to GalNAc via an α(1,4) linkage. Finally, HA is similar to CS-A but replaces GalNAc with N-acetyl-D-glucosamine (GlcNAc) and contains no sulfation (Fig. 1b ). Fig. 1: Model of glycosaminoglycan degradation by PUL CS/DS/HA . a Organisation of the PUL CS/DS/HA locus in Bacteroides thetaiotaomicron . b Schematic depiction of the activity, location and specificity of PUL CS/DS/HA encoded enzymes. Asterisk indicates structures were solved in this study. Full size image PUL CS/DS/HA structure B. theta grows on CS-A, CS-C, DS and HA and transcriptomics, on CS-C and HA, demonstrate only PUL CS/DS/HA and two additional genes, BT1596-S1_9 2S-sulf and BT4410 PL33 are upregulated [4] , [13] . PUL CS/DS/HA encodes three PLs (BT3324 PL8 , BT3328 PL29 and BT3350 PL8 ), one GH88 (BT3348 GH88 ), 2-O-sulfatases (BT3333-S1_15 6S-sulf and BT3349-S1_27 4S-sulf) , a single SusC/D-like transporter system (BT3331 susD -BT3332 susC ), a hybrid two-component sensor (BT3334 HTCS ) and two proteins of unknown function (BT3329 and BT3330). The non-PUL encoded genes, BT1596-S1_9 2S-sulf and BT4410 PL33 , encode a 2-O sulfatase and a hyaluronidase, respectively (Fig. 1a, b ). A paradigm for how PULs organise their protein apparatus has been established. A surface enzyme(s), with usually one SGBP, degrades and captures large polysaccharides/oligosaccharides at the cell surface. These partially degraded polysaccharides/oligosaccharides are transported into the periplasm through the action of the highly conserved, and critical, SusC/D-like transporter system. Small polysaccharides/large oligosaccharides transported into the periplasm are then metabolised to their constituent parts, usually monosaccharides, and transported into the cytoplasm to enter cytoplasmic metabolic pathways. Extracellular glycan binding and degradation Two genes of unknown function BT3329 and BT3330 exist within PUL CS/DS/HA . Both proteins had no enzymatic activity against any GAG substrates. However, they were shown to exhibit binding by isothermal titration calorimetry (ITC). Both proteins were able to bind all four GAGs and were thus classified as SGBPs (Supplementary Fig. 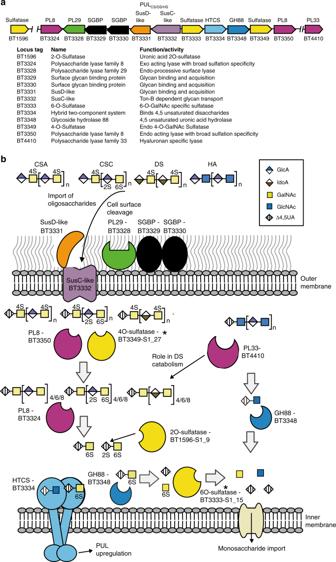Fig. 1: Model of glycosaminoglycan degradation by PULCS/DS/HA. aOrganisation of the PULCS/DS/HAlocus inBacteroides thetaiotaomicron.bSchematic depiction of the activity, location and specificity of PULCS/DS/HAencoded enzymes. Asterisk indicates structures were solved in this study. 1 and Supplementary Table 1 ). BT3329 SGBP bound to CS-A and HA with approximately ten and fourfold higher affinity than BT3330 SGBP whilst against CS-C and DS BT3329 SGBP bound with an ~100 and ~50-fold higher affinity. BT3329 SGBP but not BT3330 SGBP bound a CS oligosaccharide of DP10. BT3330 SGBP was, however, able to bind a CS oligosaccharide of DP20. The SGBPs thus differ in their polysaccharide and oligosaccharide preferences. BT3329 SGBP has the ability to bind more variably sulfated and smaller glycans than BT3330 SGBP , and displays a greater tolerance to iduronic acid (Supplementary Fig. 1 and 2a ). Both proteins were confirmed to be extracellular by immunofluorescence assays (Supplementary Fig. 2b ). BT3331 susD demonstrated a very strict substrate specificity binding only to CS-A with a measurable affinity, similar to that of BT3329 SGBP (Supplementary Table 1 ). The surface lyase, BT3328 PL29 , showed its highest enzymatic activity and affinity against CS-A > CS-C > HA and little activity on DS, differing from previous data [18] . End point assays, the total number of glycosidic bonds cleaved, followed the relationship of HA > CS-C > CS-A (Fig. 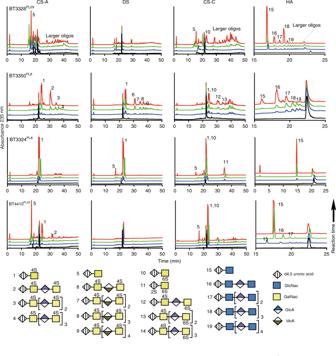Fig. 2: HPLC product profiles of the PULCS/DS/HAencoded lyases. Peaks were identified by comparison with commercially purchased standards. The black, blue, green and red lines represent 0, early, mid-point and late stages of the reaction time course for each enzyme (CS-A chondroitin sulfate A, DS dermatan sulfate, CS-C chondroitin sulfate C and HA hyaluronic acid). All reactions were carried out in 50 mM MES, pH 6.5, with 150 mM NaCl at 37 °C. 2 and Supplementary Table 2 ). This demonstrates that although O4 sulfation increases BT3328 PL29 activity on CS-A it also limits glycosidic bond access in some contexts. BT3328 PL29 was only able to cleave HA oligosaccharides with a DP ≥ 8, indicating the enzyme has at least eight subsites (Supplementary Fig. 4a ). Interestingly, BT3328 PL29 displays very similar substrate specificities to BT3331 susD which, could suggest that the proteins work closely together at the cell surface. When BT3328 PL29 was incubated with HA oligosaccharides of d.p. 12, 10 and 8, labelled at their reducing end with a fluorescent tag, a labelled trisaccharide was produced from d.p. 12 substrate and a labelled disaccharide was produced from d.p. 10 and 8 substrates. These data indicate that BT3328 PL29 cleaves glycans from the reducing end (Supplementary Fig. 2c, d and Supplementary discussion). We identified a conserved region of ~300 amino acids at the N-terminal of BT3328 PL29 and BT3329 SGBP . This region was also shared with SGBP-positioned genes from other PULs, which do not share a detectable sequence similarity downstream of this ~300 amino acid at the N-terminal region, like BT3328 PL29 and BT3329 SGBP . This might constitute a ‘spacer’ domain, not homologous but, functionally equivalent to the BACON domain found at the N-terminal region of the surface-anchored GH5 in the xyloglucan PUL [7] and in many other SGBPs. Such domains would allow extracellular proteins to extend out of the capsular envelope and/or increase their mobility. Fig. 2: HPLC product profiles of the PUL CS/DS/HA encoded lyases. Peaks were identified by comparison with commercially purchased standards. The black, blue, green and red lines represent 0, early, mid-point and late stages of the reaction time course for each enzyme (CS-A chondroitin sulfate A, DS dermatan sulfate, CS-C chondroitin sulfate C and HA hyaluronic acid). All reactions were carried out in 50 mM MES, pH 6.5, with 150 mM NaCl at 37 °C. Full size image Protein–protein interactions The interaction of the cell surface proteins with one another was assessed by Native PAGE and co-immunoprecipitation (Co-IP). Native PAGE demonstrated that BT3328 PL29 , BT3329 SGBP , BT3330 SGBP and BT3331 SusD displayed no observable interaction in vitro (Supplementary Fig. 3a, b ). Co-IP data, however, demonstrated that at the cell surface BT3328 PL29 , BT3329 SGBP and BT3330 SGBP do indeed interact (Supplementary Fig. 3c–e ). Co-IPs using anti-BT3328 PL29 and anit-BT3329 SGBP antibodies revealed the presence of both BT3329 SGBP and BT3330 SGBP in BT3328 PL29 -IP and the presence of both BT3328 PL29 and BT3330 SGBP in BT3329 SGBP -IP. When the BT3330 SGBP precipitant was analysed only BT3329 SGBP could be observed and not BT3328 PL29 . Collectively these data suggest that BT3328 PL29 , BT3329 SGBP and BT3330 SGBP interact with each other at the bacterial cell surface in vivo. This interaction requires either membrane attachment or the presence of the integral membrane protein BT3332 SusC . Periplasmic glycan degradation apparatus Biochemical analysis of the periplasmic lyases: BT3324 PL8 and BT3350 PL8 are both PL8s whilst BT4410 has recently been classified into family PL33. BT3350 PL8 is a broad specificity lyase having similar activity on CS-A, CS-C and DS but had reduced activity on HA (Supplementary Table 2 ). BT3350 PL8 displayed an endo mode of action but disaccharides were observed earlier in the reaction time course on the sulfated substrates (Fig. 2 ). End point assays revealed that BT3350 PL8 could cleave similar amounts of glycosidic linkages in CS-A and DS but around half as much in the GAGs CS-C and HA (Supplementary Table 2 ). The end products of BT3350 PL8 HA degradation are mainly of DP2, 4 and 6, with oligos of ≥DP4 making up the majority of the population (Fig. 2 ). Against CS-A the end products were mainly DP2 and DP4, whilst against CS-C and DS a greater quantity of products >DP6 were observed. Surprisingly, BT3350 PL8 was able to cleave HA oligos down to disaccharides (Supplementary Fig. 4a ). BT3324 PL8 is an exo-acting lyase releasing exclusively disaccharides from all the GAGs tested (Fig. 2 and Supplementary Fig. 4a ). BT3324 PL8 displayed its highest activity against CS-A and DS with much reduced activities against CS-C and HA. Thus, O4 sulfation is required for maximal activity. BT4410 PL33 displayed a highly endo-processive mode of action and displayed >100-fold preference for HA. End point assays showed the presence of sulfation limited substrate accessibility, consistent with BT4410 PL33 being tailored towards HA (Fig. 2 and Supplementary Table 2 ). Genetic analyses of the PUL CS/DS/HA lyases: The contribution of each lyase in GAG metabolism was further assessed through growth experiments with single, double and triple genetic mutants. Using CS-A and CS-C as the substrate, we observed that individual PL mutants exhibited very little evidence of growth defects; Δbt3324 exhibited a slight defect in growth rate on CS-A (Fig. 3a ). The Δbt3350/Δbt4410 showed a stronger phenotype than Δbt3324/Δbt3350 on CS-A, whilst on CS-C both mutants exhibited the same level of defect. This is due to O6 and/or O2 sulfation in CS-C being inhibitory to BT4410 PL33 . Whilst for CS-A the endo 4S sulfatase, BT3349-S1_27 4S-sulf (see ‘O-sulfatases’ section), is able to remove 4S sulfation thus allowing enhanced activity of BT4410 PL33 on CS-A (Further detail in Supplementary discussion). The double-mutant Δbt3324/Δbt4410 showed extremely limited or no growth on all substrates, comparable with the triple-mutant Δbt3324/Δbt3350/Δbt4410 (Fig. 3a ). The Δbt3324/Δbt4410 mutant was previously shown to have drastically reduced BT3333-S1_15 6S-sulf mRNA levels in the presence of CS [13] , thus, BT3350 PL8 alone cannot generate disaccharides at a significant rate as to upregulate the PUL. BT3350 PL8 must, therefore, work in conjunction with BT3324 PL8 and BT4410 PL33 to complete GAG catabolism to their disaccharide repeating units. These data are consistent with BT3350 PL8 generating new non-reducing ends for BT3324 PL8 and BT4410 PL33 to act on, demonstrating an endo–exo synergy as commonly observed in other glycan-degrading systems. When HA is the substrate, all mutants that show a defect involved the deletion of BT4410 PL33 . The Δbt4410 mutant by itself was sufficient to cause a severe growth defect, whilst the Δbt3324/Δbt3350 mutant showed only a minor defect, reinforcing the critical role of BT4410 PL33 as a hyaluronan specific lyase (Fig. 3a ). When DS is the growth substrate, loss of any periplasmic lyase alone is sufficient to cause a significant defect, but loss of either BT4410 PL33 or BT3350 PL8 is particularly severe (Fig. 3a ). Both enzymes have endo character indicating that the ability to cleave linkages internally in DS is critical to its breakdown by B. theta . All double mutants failed to grow at all on DS (Fig. 3a ). Fig. 3: Analysis of genetic knockouts and their effect on glycosaminoglycan metabolism. a Growth of genetic knockouts on glycosaminoglycan substrates (CS-A chondroitin sulfate A, DS dermatan sulfate, CS-C chondroitin sulfate C and HA hyaluronic acid); b TLC analysis of purified oligosaccharide (X), left behind in media from Δbt3324 growths, against PUL CS/DS/HA encoded lyases; c HPLC analysis of X treated with BT3324 PL8 . Data represent technical triplicates and source data are provided in the source data file labelled as mutant growths. Full size image Analyses of spent supernatants from genetic mutants: Analysis of spent supernatants from mutant growths revealed that the Δbt3324 mutant, produced a unique product. This substrate was purified and treated with the different lyases; only BT3324 PL8 showed activity (Fig. 3b ). The products were analysed by HPLC and two peaks were identified as UA2S-GalNAc6S disaccharide and either UA-GalNAc4S or UA-GalNAc6S in a ratio of 3:1 (Fig. 3c ). The accumulation of this substrate reveals that BT3324 PL8 is the only enzyme in B. theta capable of cleaving regions within CS-C enriched in 2S sulfation. O-Sulfatases PUL CS/DS/HA encodes two O sulfatases belonging to the sulfatase subfamilies S1_27 and S1_15, the endo 4S sulfatase BT3349-S1_27 4S-sulf and the exo-acting 6S sulfatase BT3333-S1_15 6S-sulf , as classified by the sulfatlas database [19] . BT1596-S1_9 2S-sulf is located outside the PUL and belongs to subfamily S1_9. BT3349-S1_27 4S-sulf and BT1596-S1_9 2S-sulf are active on all O4 and O2 sulfated CS disaccharides, respectively. This is consistent with previous work on these subfamilies [20] . Whilst BT3333-S1_15 6S-sulf was only active on GalNAc6S and is the first member to be functionally and structurally characterised within the S1_15 subfamily (Supplementary Fig. 4b, c ). 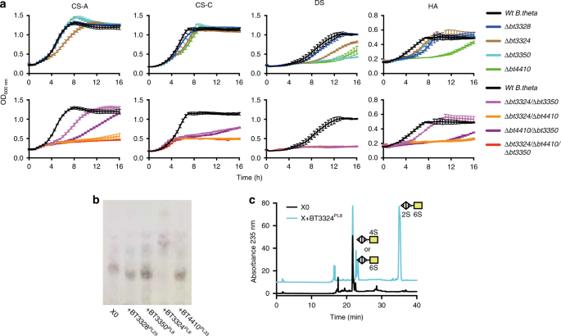Fig. 3: Analysis of genetic knockouts and their effect on glycosaminoglycan metabolism. aGrowth of genetic knockouts on glycosaminoglycan substrates (CS-A chondroitin sulfate A, DS dermatan sulfate, CS-C chondroitin sulfate C and HA hyaluronic acid);bTLC analysis of purified oligosaccharide (X), left behind in media fromΔbt3324growths, against PULCS/DS/HAencoded lyases;cHPLC analysis of X treated with BT3324PL8. Data represent technical triplicates and source data are provided in the source data file labelled as mutant growths. BT3349-S1_27 4S-sulf contains an SpII signal peptide (Supplementary Table 3 ) and, due to its endo mode of action, it was hypothesised that the enzyme may be attached to the extracellular surface. Measures of the enzymatic activity at the cell surface by whole-cell assays (see ‘Methods’) did not result in any degradation of Δ4,5UA-GalNAc4S, a substrate for BT3349-S1_27 4S-sulf , even after an incubation time of 16 h. However, when the cells were sonicated and the disaccharide incubated with the CFE, Δ4,5UA-GalNAc4S was completely degraded within 1 h (Supplementary Fig. 4d ). This confirms BT3349-S1_27 4S-sulf is a periplasmic enzyme. BT3333-S1_15 6S-sulf also contains an SpII signal peptide but whole-cell assays, using GalNAc6S, indicate that BT3333-S1_15 6S-sulf is periplasmic (Supplementary Fig. 4d ). This is consistent with the requirement for the periplasmic BT3348 GH88 to produce its GalNAc6S substrate (Supplementary Fig. 4d ). Crystal structures of BT3349-S1_27 4S-sulf and BT3333-S1_15 6S-sulf : Both enzymes are α/β proteins, composed of two domains, a larger N-terminal domain and a smaller C-terminal ‘sub-domain’ as is typical of formylglycine sulfatases [21] . An inactive form of BT3349-S1_27 4S-sulf was crystallised with a CS-A tetrasaccharide, but only a trisaccharide of Δ4,5UA-GalNAc4S-GlcA could be modelled (Fig. 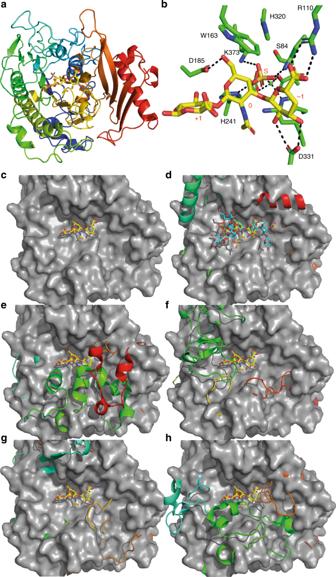Fig. 4: Structural depictions of BT3349-S1_274Sand its comparison with other endo and exo sulfatases. aCartoon representation of BT3349-S1_274S-sulframped blue to red from its N- to C-terminus;bstick representation of binding site interactions with the protein in green and the bound trisaccharide yellow;csurface representation of BT3349-S1_274S-sulfshowing how the +1 and −1 ends of the trisaccharide are free to be extended;doverlays of surface representations of BT3349-S1_274S-sulfand a cartoon of the marine endo 4S ι-carrageenan sulfatase (PsS1_19A). CS and ι-carrageenan oligosaccharides are shown in yellow and cyan, respectively.eOverlay of a surface of BT3349-S1_274S-sulfwith a cartoon of the exo-sulfatase BT1596-S1_92S-sulf.fOverlay of a surface of BT3349-S1_274S-sulfwith a cartoon of the exo-sulfatase BT3333-S1_156S-sulf.gOverlay of a surface of BT3349-S1_274S-sulfwith a cartoon of the human exo-sulfatase 1FSU4S-sulf.hOverlay of a surface of BT3349-S1_274S-sulfwith a cartoon of the human exo-sulfatase 5FQL2S-sulf. All cartoon representations are ramped blue to red from their N- to C-terminus. 4a, b , Supplementary Fig. 5a ). Subsite nomenclature for carbohydrate sulfatases is such that an S site denotes the position of the labile sulfate, which is attached to a 0 subsite sugar. Additional subsites then increase in number toward the reducing end of the glycan, i.e. +1, +2, etc., and decrease in number toward the non-reducing end of the glycan, i.e. −1, −2, etc [22] . Electron density for the −1, 0 and S subsites was well ordered whilst the +1 GlcA was partially disordered and makes no interactions with the protein. 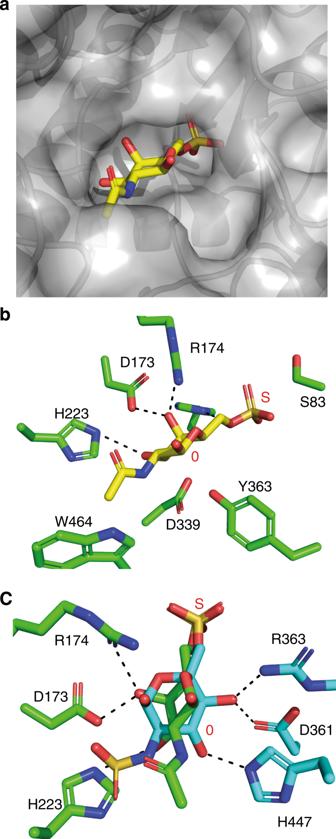Fig. 5: Structural depictions of BT3333-S1_156S-sulfand it comparison with BT46566S-sulf. aA close up of a surface representation showing the pocket topography of BT3333-S1_156S-sulf;bstick representations of the binding site interactions with the protein in green and GalNAc6S in yellow;coverlay of BT3333-S1_156S-sulfin complex with GalNAc6S (green) and BT4656-s1-116S-sulfin complex GlcNAc6S (cyan). A detailed description of the mutants is provided in the supplementary discussion (Supplementary Table 5 and Supplementary Fig. 5e ). The endo activity of BT3349-S1_27 4S-sulf is conferred by an ‘opening up’ of either side of the 0 subsite, allowing glycan extension in both the +1 and −1 direction. Structural comparison of HGM, marine and human carbohydrate sulfatases reveals that the linker between β-strand 4 and α-helix 5 is extended, and/or alterations of the C-terminal subdomain (Fig. 4c–h ) commonly occur in the exo sulfatases, precluding endo activity. In BT3333-S1_15 6S-sulf , however, occlusion of potential positive subsites is achieved by an insertion between β-strand 3 and α-helix 4. These features would also prevent extension of the sugar chain beyond the 0 subsite in the endo sulfatases. Fig. 4: Structural depictions of BT3349-S1_27 4S and its comparison with other endo and exo sulfatases. a Cartoon representation of BT3349-S1_27 4S-sulf ramped blue to red from its N- to C-terminus; b stick representation of binding site interactions with the protein in green and the bound trisaccharide yellow; c surface representation of BT3349-S1_27 4S-sulf showing how the +1 and −1 ends of the trisaccharide are free to be extended; d overlays of surface representations of BT3349-S1_27 4S-sulf and a cartoon of the marine endo 4S ι-carrageenan sulfatase (PsS1_19A). CS and ι-carrageenan oligosaccharides are shown in yellow and cyan, respectively. e Overlay of a surface of BT3349-S1_27 4S-sulf with a cartoon of the exo-sulfatase BT1596-S1_9 2S-sulf . f Overlay of a surface of BT3349-S1_27 4S-sulf with a cartoon of the exo-sulfatase BT3333-S1_15 6S-sulf . g Overlay of a surface of BT3349-S1_27 4S-sulf with a cartoon of the human exo-sulfatase 1FSU 4S-sulf . h Overlay of a surface of BT3349-S1_27 4S-sulf with a cartoon of the human exo-sulfatase 5FQL 2S-sulf . All cartoon representations are ramped blue to red from their N- to C-terminus. Full size image The structure of BT3333-S1_15 6S-sulf was solved in complex with GalNAc6S and displays a pocket topology (Fig. 5a , Supplementary Fig. 5b ). The 0 subsite is made up primarily of polar interactions (Fig. 5b ). The axial O4 of the GalNAc (the unique difference of Gal versus Glc-configured substrates, the latter having an equatorial O4) coordinates with O δ 2 of D173 and NH1 of R174 (for further interactions see Supplementary discussion). These interactions probably drive the specificity for GalNAc versus GlcNAc substrates. R174 also coordinates with O1 and the endocyclic ring oxygen through NH 2 whilst O3 interacts with the Nε2 of H225A (Fig. 5b ). Comparing overlays of BT3333-S1_15 6S-sulf with BT4656-S1_11 6S-sulf , the GlcNAc6S sulfatase encoded by PUL Hep , reveals that the two substrates bind perpendicular to one another and thus no interactions are spatially conserved (Fig. 5c ). Despite this both enzymes use an Asp and Arg to bind O4 and a His to co-ordinate O3. In BT3333-S1_15 6S-sulf these residues are from the N-terminal side of the protein (D173, R174 and H225) whilst in BT4656-S1_11 6S-sulf they are from the C-terminal side of the protein (D361, R363 and H447). In addition, when compared with GALNS (4FDJ), the human 6S GalNAc sulfatase, there is no conservation of the sugar-binding residues between the two proteins (Supplementary Fig. 5c–e ). Currently no substrate complex of GALNS exists and the specificity determinants remain undescribed. Fig. 5: Structural depictions of BT3333-S1_15 6S-sulf and it comparison with BT4656 6S-sulf . a A close up of a surface representation showing the pocket topography of BT3333-S1_15 6S-sulf ; b stick representations of the binding site interactions with the protein in green and GalNAc6S in yellow; c overlay of BT3333-S1_15 6S-sulf in complex with GalNAc6S (green) and BT4656-s1-11 6S-sulf in complex GlcNAc6S (cyan). Full size image GH88 enzyme The BT3348 GH88 is an essential enzyme for CS metabolism [13] . BT3348 GH88 showed a similar catalytic efficiency against Δ4,5UA-GalNAc, Δ4,5UA-GalNAc6S and Δ4,5UA-GlcNAc but was inactive against Δ4,5UA2S-GalNAc, Δ4,5UA-GalNAc4S, Δ4,5UA-GalNAc4S6S and Δ4,5UA2S-GalNAc4S6S (all β1,3 linked). BT3348 GH88 was also inactive on the β1,4 linked heparin disaccharide Δ4,5UA-GlcNAc (Supplementary Table 5 ). BT3348 GH88 can tolerate O6 sulfation but not O2 or O4 sulfation, and is specific for the β1,3 linkage but has no preference for GlcNAc or GalNAc at its +1 subsite. Growth and bioinformatic analyses of gut Bacteroides species Eleven Bacteroides species were grown on each GAG as sole carbon source and classified as either strong, intermediate or non-utilisers. For CS-A and CS-C B. theta , B. ovatus , B. eggerthii , B. xylanisolvens and B. plebeius were all strong utilisers whilst B. caccae , B. cellulosilyticus , and B. intestinalis demonstrated intermediate growth. When DS was the substrate there was a shift in classifications compared with CS-A and CS-C. B. eggerthii and B. plebeius switched to being non-utilisers whilst B. intestinalis was classified as a strong utiliser. When HA was the substrate B. ovatus and B. eggerthii out performed all other strains. Only B. theta grew as fast but was classified as intermediate due to a ~20% lower final OD 600 nm (Fig. 6 ). Fig. 6: Growth curves of 11 bacteroides species on CS-A, DS, CS-C and HA. The different species were divided into strong, intermediate and non-utilisers based on analysis of growth curve rates and final optical densities. Data represent technical triplicates and source data are provided in the source data file labelled as strain growths. Full size image Orthologous proteins were searched to identify PUL CS/DS/HA relatives in the eleven species. The three strains B. vulgatus , B. dorei and B. fragilis lack PUL CS/DS/HA and only harbour a BT3348 GH88 orthologue (and a separated BT4410 PL33 in B. fragilis ). Consistently, all three showed no growth on any GAGs. We observed BT3328 PL29 -BT3330 SGBP were more rapidly diverging and completely lost in B. cellulosilyticus , B. intestinalis and B. eggerthii . However, no impact on growth was observed, consistent with Δbt3328 mutant growth data. The only genetic differences with potential growth impacts were the loss of BT4410 PL33 orthologues in both B. eggerthii and B. plebeius (which additionally lacks a BT3350 PL8 orthologue). The importance of BT4410 PL33 for B. theta growth on DS and HA (i) explains the switch of B. eggerthii and B. plebeius from strong utilisers on CS-A and CS-C to non-utilisers on DS; (ii) suggests that alternative pathways for HA catabolism exist in these organisms compared with B. theta . B. eggerthii notably outcompeted most other strains on CS-A, CS-C and HA. This could mean members of the PL35 (BACPLE_02279, BACEGG_01448) or PL37 (BACEGG_00231) which are active on GAGs [16] , [23] and not present in B. theta , are contributing to this enhanced growth. Comparative genomic analyses on a thousand Bacteroidetes species revealed that PUL CS/DS/HA is largely associated with the Bacteroides genus but not ubiquitous. Different sections are variably conserved and may have accessory interest, like the aforementioned BT3328 PL29 -BT3330 SGBP region (Supplementary Fig. 6 and Supplementary Table 5 ). Also, many insertions are observed which separate the PUL elements into several islands, without impairing the PUL activity, according to growth data. Examples span from the three-gene insertion specific to B. theta strains (BT3344-BT3347 that includes an unrelated susCD pair) to hundreds of genes separating B. plebeius orthologues into three genomic regions (Supplementary Fig. 6 ). Thus, orthologue conservation is more relevant over a tight organisation when predicting growth. Searches beyond the human gut Bacteroides genus reveal species having all required orthologues for growth in the Chitinophaga , Cytophaga and Sphingobacteria classes (some from human skin, chicken gut and soil environments). Notably, a tightly packed PUL was found in Propebela bergensis that even incorporates BT4410 PL33 within the core PUL (Supplementary Fig. 6 ). PUL CS/DS/HA performs a highly co-ordinated degradation of GAGs but in a contrasting way to the previously described PUL Hep , which degraded H/HS. PUL Hep encodes four PLs all of which displayed significant processivity with variable sulfation tolerances [24] . PUL CS/DS/HA , however, utilises endo–exo synergy in the periplasm between BT3350 PL8 and BT3324 PL8 for the degradation of CS-A, CS-C and DS. The PUL also deploys an endo-acting O4 sulfatase, BT3349-S1_27 4S-sulf , the rationale behind its endo mode of action, however, is not obvious. BT3349-S1_27 4S-sulf may enable BT4410 PL33 to contribute to the degradation of CS-A and DS, where O4 sulfation would be inhibitory. A surprising finding was the important role BT4410 PL33 plays in DS metabolism within the Bacteroides genus, a result that could not be predicted. The anchoring of BT3349-S1_27 4S-sulf to the periplasmic side of the membrane may localise it close to the SusC and where it could remove O4 sulfation as glycans enter the periplasm. Alternatively, it could be localised close to BT3334 HTCS and BT3348 GH88 , neither of which can utilise O4 sulfated disaccharides [13] and are also membrane associated. This may allow O4 sulfated disaccharides to be desulfated close to the HTCS before BT3348 GH88 can degrade them. BT1596-S1_9 2S -sulf must remove any 2S sulfation present for BT3348 GH88 to act. BT3333-S1_15 6S-sulf then removes the O6 sulfation of GalNAc leaving the final degradation products as GalNac and 4-deoxy-L-threo-5-hexosulose-uronate. For HA metabolism BT4410 PL33 is the only lyase required due to its endo-processive mode of action, and after BT3348 GH88 has acted the final products would be GlcNAc and 4-deoxy-L-threo-5-hexosulose-uronate. 4-deoxy-L-threo-5-hexosulose-uronate is able to feed directly into metabolism in the cytoplasm [25] whilst both GlcNAc and GalNAc require phosphorylation before further metabolism. In contrast to PUL Hep , which encodes the GlcNAc kinase BT4654 ROK , PUL CS/DS/HA does not encode for any kinases. Therefore, phosphorylation of GalNAc and GlcNAc, must be completed by constitutively active kinases. Support for a constitutively active GlcNAc kinase is that deletion of BT4654 ROK in PUL Hep has no growth defect on H/HS [24] . In addition, no differentially expressed kinases are observed during CS growth. Although the extracellular glycan apparatus appears to confer no advantage in mono-cultured systems, it may be important in a multi-organism, competitive, environment. When B. theta, B. caccae and B. cellulosilyticus were co-cultured on CS for 5 days it was observed that B. cellulosilyticus CFUs were ≤100-fold lower than B. theta and B. caccae and ≤100 than B. cellulosilyticus when mono-cultured [26] . B. cellulosilyticus lacks any surface glycan apparatus whilst it is present in both B. theta and B. caccae . Goodman et al. [27] identified, through transposon mutagenesis, genes in B. theta which were important for colonisation of the mouse gut. Strains with insertion in bt3348 showed a marked decrease in output compared with input. In addition, when mice were colonised with an artificial microbiome of multiple Bacteroidetes species (including transposon mutagenised B. theta strains), B. theta strains with insertions in bt3330 and BT3349-S1_27 were much reduced in bacterial number compared with monocolonized mice. Thus, CS, DS and HA metabolism are under increased selection pressure in a competitive environment with other Bacteroidetes species. Conversely, bt3328 mutants showed increased bacterial numbers, compared with monocolonized mice, when colonised with other Bacteroidetes, Firmicutes and Actinobacteria. Indomethacin release, in the gut, from cross-linked CS is dependent upon biodegradation by the caecal contents [28] . The detailed biochemical analysis of the extracellular glycan apparatus in this study may facilitate strategies to more tightly control drug release to the digestive tract using cross-linked CS. The structural data of BT3349-S1_27 4S-sulf shows how endo-sulfatase activity has evolved and could be used to predict/guide engineering of sulfatase function. The active site of BT3333-S1_15 6S-sulf reveals the specificity determinants for Gal over Glc-configured substrates when compared with the GlcNAc6S sulfatase BT4656-S1-11 6S-sulf . These data highlight how much more highly variable the active sites of related sulfatase are than could be predicted from the nature of their respective substrates. The knowledge of the highly variable nature of the glycone-binding site of sulfatases may help design future glycosulfate-specific inhibitors. This is of timely relevance because of the recently revealed role of sulfatase action in eliciting colitis in a colitis sensitive mouse model [17] . The data presented here reveal how the HGM has evolved a core GAG utilisation machinery (PUL CS/DS/HA ) to target diverse GAGs in the human gut. PUL CS/DS/HA components included orphan, physically connected and constitutively active genes with complementary and in some cases unique activities which together enable the complete metabolism of diverse GAGs. PUL CS/DS/HA components are widely conserved in Bacteroides and thus presents a general model of CS, DS and HA metabolism, which can be applied to other members of the HGM. Sources of carbohydrates . Carbohydrates were from Sigma, carbosynth or Dextra Laboratories. All other chemical reagents were purchased from Sigma. Bacteroides culture and genetic manipulation : Various Bacteroides strains and B. theta VPI-5482 were cultured anaerobically in a Whitley A35 Workstation (Don Whitley) at 37 °C in either tryptone yeast extract glucose medium or minimal medium (MM) containing GAGs (described below). B. theta strains containing specific gene deletions or inactivated versions of enzymes were made by counter selectable allelic exchange as described below [18] . All genetic mutants, except Δbt3328 , were provided by Dr Guy E. Townsend and Prof. Eduardo Groisman [13] . The in frame mutants were generated using counter selectable allelic exchange [29] . Briefly, 1-kb fragments either side of the target gene were cloned, ‘stitched together’ by PCR, and ligated into the pExchange plasmid using SalI/XbaI sites. This recombinant plasmid was then conjugated into a tdk − version of B. theta (referred to as  wildtype (WT) in this study) using the S17-1 λ pir Escherichia coli strain. Initial homologous recombination, plasmid insertion, is selected for using erythromycin resistance. Then a second low-frequency recombination event, exclusion of the pExchange plasmid from the genome, is selected for using FUdR containing plates. In frame deletion mutants were detected and checked using PCR and sequencing. Insertional mutations were constructed by cloning a 750-bp sequence from the gene to be disrupted into the pKNOCK tet vector, followed by its introduction into the B. theta chromosome [30] . Growth of the WT and mutants was measured on glycans by mixing the autoclave-sterilised polysaccharides (0.5% final) with minimal media (per 100 ml was: 0.1 g of Ammonium sulfate and sodium carbonate, 0.05 g cysteine, 10 ml 1 M potassium phosphate pH 7.2, 0.1 ml of 1 mg ml −1 vitamin K, 1 ml of 0.4 mg ml −1 iron sulfate, 0.4 ml of 0.25 mg ml resazurin, 0.05 ml of 0.01 mg ml −1 vitamin B12 and 5 ml of mineral salts for defined media) and monitoring growth continuously in 96-well plates using a Biotek Epoch plate reader. Growth curves presented are averages of three technical replicates. Co-immunoprecipitation and western blotting : Bacterial cells were collected in the mid-exponential phase and bacterial pellets were resuspended in the lysis buffer (50 mm Tris, pH 7.5, 150 mm NaCl, 0.2 mm Na 3 VO 4 , 1% Nonidet P-40 alternative, 1 mm PMSF, 1 mm DTT, and 1× protease inhibitors (Roche Applied Science)). Lysates were sonicated followed by incubation with 1 μg of antibodies as indicated for 16 h at 4 °C, antibodies were pulled down using protein G-Sepharose beads. Samples were then run on 12.5% SDS-PAGE gels, then transferred to a nitrocellulose membrane using standard buffers. Both primary and secondary antibodies were used as 1/1000 dilutions in 5% milk powder. The secondary antibody was mouse anti-rabbit IgG-HRP (sc-2357). Normal mouse IgG (sc-2025) was used as a negative control. Both antibodies were purchased from santa-cruz. Mi croscopy : GAG grown cells were harvested at mid-exponential phase and fixed for 90 min in formalin (10% formaldehyde in PBS buffer). Primary Ab was incubated 1/500 for 2 h at room temperature (RT), followed by incubation with the secondary Ab (Santa Cruz goat anti-rabbit FITC) at 1/500 at RT for 1 h. Cells were immobilised for the microscopy by transfer on 1.2% agarose/H 2 O pads. Fluorescence microscopy was carried out with Nikon Eclipse Ti equipped with Nikon Plan Apo 100×/1.40 NA phase contrast objective, Prime sCMOS camera (Teledyne Photometrics) and Lambda LS Xenon-arc lamp (Sutter Instruments), and Chroma 49002 filter set (Chroma Technology). Images were acquired with Metamorph 7.7 (Molecular Devices) and analysed with Fiji [31] . Whole-cell assays . Whole-cell assays are a direct readout of cell surface activity. After washing with PBS there is no longer any sugar transport by the TonB dependent SuSC transporter. Therefore, product profiles and activities of surface enzymes can be assessed. B. theta was grown in 5 mL MM with 1% (wt/vol) appropriate GAG as the sole carbon source to mid-exponential phase in glass test tubes. Cells were harvested by centrifugation at 5000 × g for 10 min at RT and washed in 5 mL PBS (pH 7.2) before being resuspended in 1 mL PBS. Washed cells were assayed against 10 mg mL −1 of the appropriate substrate at 37 °C for up to 24 h. Assays were analysed by thin layer chromatography (TLC), and 2 μL each sample was spotted onto silica plates and resolved in butanol:acetic acid:water (2:1:1) running buffer. The plates were dried, and the sugars were visualised using diphenylamine stain. Recombinant protein production . Genes were amplified by PCR using the appropriate primers and the amplified DNA cloned in pET28a using BamHI/XhoI or NheI/XhoI restriction sites generating constructs with either N- or C-terminal His 6 tags (Supplementary Table 7 ). Recombinant genes were expressed in E. coli strains BL21 (DE3) or TUNER (Novagen), containing the appropriate recombinant plasmid, and cultured to mid-exponential phase in LB supplemented with 50 μg/mL kanamycin at 37 °C and 180 rpm. Cells were then cooled to 16 °C, and recombinant gene expression was induced by the addition of 0.1 mM isopropyl β-D-1-thiogalactopyranoside; cells were cultured for another 16 h at 16 °C and 180 rpm. The cells were then centrifuged at 5000 × g and resuspended in 20 mM Hepes, pH 7.4, with 500 mM NaCl before being sonicated on ice. Recombinant protein was then purified by immobilised metal ion affinity chromatography using a cobalt-based matrix (Talon, Clontech) and eluted with 100 mM imidazole. For the proteins selected for structural studies (BT3333-S1_15 6S-sulf and BT3349-S1_27 4S-sulf ), another step of size-exclusion chromatography was performed using a Superdex 16/60 S200 column (GE Healthcare), with 10 mM Hepes, pH 7.5, and 150 mM NaCl as the eluent, and they were judged to be ≥95% pure by SDS-PAGE. Protein concentrations were determined by measuring absorbance at 280 nm using the molar extinction coefficient calculated by ProtParam on the ExPasy server ( web.expasy.org/protparam/ ). Isothermal Calorimetry (ITC) . The affinity of BT3329 SGBP , BT3330 SGBP and BT3331 SusD for oligo- and polysaccharides was quantified by ITC using a Microcal VP calorimeter. The protein sample (50 μM), stirred at 394 rpm in a 1.4-mL reaction cell, was injected with 26 × 10-μL aliquots of ligand. Titrations were carried out in 50 mM Tris-HCl buffer, pH 8.0, at 25 °C. Integrated binding heats minus dilution heat controls were fit to a single set of sites binding model to derive K A , Δ H and n (number of binding sites on each molecule of protein) using Microcal Origin v7.0. The molar concentration of binding sites present in polysaccharides for BT3329 SGBP was determined by altering the concentration of ligand used for regression of the isotherm until the fit yielded a value of 1 for n . For BT3330 SGBP and BT3331 SusD n was fixed to 1 and a ligand concentration of 2 mM was used. Enzyme assays . All assays, unless stated, were carried out in 50 mM MES, pH 6.0, or Bis-Tris propane, pH 6.5, with 150 mM NaCl at 37 °C. PL activity was monitored continuously at A 235 nm by the formation of the carbon double bond generated through the enzymes beta elimination mechanism of action. BT3334 GH88 glucuronyl hydrolase activity was determined by monitoring loss of signal at A 235nm . The kinetic parameters of BT3349-S1_27 4S were monitored via a continuous linked assay using BT3334 GH88 and UA-GalNAc4S as the substrate. BT3334 GH88 will only hydrolyse UA-GalNAc4S after it has been converted to UA-GalNAc by BT3349-S1_27 4S-sulf and thus loss of sulfation can be monitored indirectly by loss of signal at A 235nm caused by BT3334 GH88 hydrolysing any UA-GalNAc produced. The ability of BT3333-S1_15 6S-sulf , BT3349-S1_27 4S-sulf and BT1596-S1_9 2S-sulf to remove O 2 , O 4 and O 6 sulfation, respectively, from unsaturated CS disaccharides was also monitored qualitatively by TLC. Reaction profiles of PLs and sulfatase digestion of GAGs were monitored by HPAEC using an AD25 or a VWD, Thermofisher, absorbance detector at A 235nm to detect the carbon–carbon double bond products, with H 2 O, pH 3.5, as the eluent and a second eluent of H 2 O with 3 M NaCl used to generate a linear NaCl gradient to 100% over 90 min. All enzymatic assays were performed in technical triplicate. Labelling of glycans : Labelling with 2-aminobenzamide acid (2-AB) was performed using the ludgerTag 2-AB glycan labelling kit. Briefly, DMSO was added to acetic acid in a 0.75:1 ratio and 100 μl added to 5 mg of 2-AB. This mixture is then added to the reductant sodium cyanoborohydride and when fully dissolved 5 μl was added to 50 nmol of dried HA dodecasaccharide. The reaction was left at 65 °C for ~3 h. After labelling samples were cleaned up using the provided spin columns. Labelling of HA octasaccharide and decasaccharide was carried out by creating a saturated solution of 7-aminonapthalene-1,3-disulfonic acid (ANDSA) in formamide and mixing this with 500 μg of dried glycan. The mixture was left overnight at RT and the labelled glycans used the next day in a 1/5 dilution versus enzyme buffer. Saccharides labelled using the UV fluorescent tag, ANDSA were run on 33% acrylamide tris-acetate gels with tris-MES running buffer. Gels were viewed after removal from the glass plates on a UV transilluminator [32] . Crystallisation of BT3333-S1_15 6S-sulf and BT3349-S1_27 4S-sulf . After purification, BT3333-S1_15 6S-sulf and BT3349-S1_27 4S-sulf were carried forward in the same eluent as used for the size-exclusion chromatography. All proteins were then concentrated in centrifugal concentrators with a molecular mass cutoff of 30 kDa. Sparse matrix screens were set up in 96-well sitting drop TTP Labtech plates (400-nL drops). Initial BT3333-S1_15 6S-sulf apo crystals were obtained at 20 mg/mL in 20% PEG 3350 and KCl. For BT3349-S1_27 4S-sulf ligand-bound initial hits were obtained at 20 mg mL −1 in 20% PEG 3350 and 0.2 M K acetate. BT3349-S1_27 4S-sulf crystals were soaked overnight with 10 mM of a CS tetrasaccharide prior to fishing. BT3333-S1_15 6S-sulf ligand-bound forms were crystallised at 20 mg mL −1 with 10 mM GlaNAc6S in 30% PEG 4000, 200 mM MgCl 2 , and 0.1 M Tris, pH 8.5. All crystals were cryo-cooled with the addition of 20% PEG 400. Data were collected at Diamond Light Source (Oxford) on beamlines I24 and I04-1 (0.98 Å) at 100 K. The data were integrated with XDS [33] and scaled with Aimless [34] , [35] . Five percent of observations were randomly selected for the R free set. The phase problem was solved by molecular replacement using the program automated molecular replacement server Balbes [36] for BT3349-S1_27 4S-sulf . The phase problem for BT3333-S1_15 6S-sulf was initially solved using Molrep [37] and BT1624 (unpublished structure) as the search model. This gave a partial solution, which could not be fully solved due to tNCS and/or twinning. A good enough model of BT3333-S1_15 6S-sulf was constructed to be used to solve the phase problem for subsequent collected data, which showed no tNCS and/or twinning defects. Models underwent recursive cycles of model building in Coot [38] and refinement cycles in Refmac5 [39] . The models were validated using Coot [38] and MolProbity [40] . Structural Figures were made using Pymol (the PyMOL Molecular graphics system, Version 2.0 Schrodinger, LLC) and all other programmes used were from the CCP4 suite [41] . 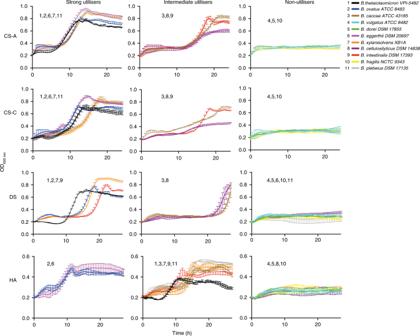Fig. 6: Growth curves of 11 bacteroides species on CS-A, DS, CS-C and HA. The different species were divided into strong, intermediate and non-utilisers based on analysis of growth curve rates and final optical densities. Data represent technical triplicates and source data are provided in the source data file labelled as strain growths. The data processing and refinement statistics are reported in Supplementary Table 6 . Site-directed mutagenesis . Site-directed mutagenesis was conducted using the PCR-based QuikChange kit (Stratagene) according to the manufacturer’s instructions using the appropriate plasmid as the template and appropriate primer pairs. Comparative genomics analysis . Similar PULs were searched in >900 Bacteroidetes genomes as follows. First, we identified orthologous proteins to PUL CS/DS/HA based on reciprocal best BlastP results between B. theta and each species. Orthologous proteins were mapped to their PUL predictions in PULDB to identify loci gathering several orthologues. For the 11 species tested for growth, PUL predictions were manually refined (enlarged) for boundaries to cover the whole PUL CS/DS/HA region which included variable insertions between the core operon and BT3324 or BT3349-S1_27-BT3350 orthologues. Reporting summary Further information on research design is available in the Nature Research Reporting Summary linked to this article.